Mst1 regulates integrin-dependent thymocyte trafficking and antigen recognition in the thymus Thymocyte trafficking has an important role in thymic selection. Here we show that the Hippo homologue Mst1 is required for thymocyte migration and antigen recognition by LFA-1 and ICAM-1 within the medulla. Using two-photon imaging of thymic tissues, we found that highly motile mature thymocytes arrest and are activated in the vicinity of rare populations of Aire + ICAM-1 hi medullary thymic epithelia in a negatively selecting environment. Notably, Mst1 deficiency or blocking the cell adhesion molecules LFA-1 and ICAM-1 results in inefficient migration and antigen recognition of CD4 + thymocytes within the medulla. Consistent with these defects, thymocyte selection is impaired in Mst1 −/− mice, which display T cell-dependent inflammatory infiltrates in multiple organs and develop autoantibodies. Our results suggest that Mst1 has a key role in regulating thymocyte self-antigen recognition in the medulla. The dynamic behaviour of developing T-cell precursors in the thymus is important for proper development and self-reactivity screening before T cells exit the thymus [1] , [2] . Immature CD4 + CD8 + double-positive (DP) cells expressing a stochastically rearranged T-cell receptor (TCR), localize throughout the cortex and are positively selected by low-avidity interactions with self-peptide/MHC on cortical thymic epithelial cells (cTECs). Then, these positively selected thymocytes become single-positive (SP) cells and localize primarily in the medulla, where SP cells that strongly interact with self-antigens are deleted by negative selection. Autoimmune regulator (Aire) is expressed in medullary thymic epithelial cells (mTECs) and regulates the expression of tissue-restricted antigen (TRA) in the medulla [3] , [4] . Mutations in Aire cause loss of TRA expression in the thymus and a failure to delete organ-specific T cells [5] , [6] , leading to multiple organ autoimmunity in humans and mice [7] . Two-photon imaging has been used to show that these selection processes are associated with changes in the migration behaviour of thymocytes [8] , [9] , [10] . In the cortex, DP thymocytes crawl and transiently interact with cortical thymic epithelial cells. After positive selection, thymocytes move much faster and with directional migration towards the medulla. The entry and migration of thymocytes in the medulla is regulated by chemotactic signals and specific migratory substrates [11] . Pertussis toxin-sensitive signalling, including signalling through the chemokine receptor CCR7 on SP cells, provides the critical signal to enter and accumulate in the medulla [11] . GIT2 −/− DP cells are hyper-responsive to chemotactic cues, which bias localization in the cortex, leading to perturbations in the positive selection process [12] . CCR7-deficient mice develop autoimmunity because of defective negative selection [13] , [14] , [15] , [16] . However, the mechanisms by which thymocyte trafficking controls these selection processes are not well understood. Mst1 (also known as Stk4 ) is the mammalian homologue of Drosophila Hpo , which controls organ size by negatively regulating cell proliferation and apoptosis [17] , [18] . Mst1 interacts with a Rap1-binding protein RAPL (Rassf5c) and transmits Rap1-RAPL signals to induce polarized morphology and integrin-dependent lymphocyte adhesion by TCR and chemokines [19] . Mst1-deficient mice generated by gene-targeted or -trapped Mst1 exhibit hypoplastic lymphoid organs because of defective lymphocyte trafficking [20] , [21] , [22] . Thymocyte egress in Mst1-deficient mice is also impaired, leading to a modest increase in mature thymocytes [20] , [21] . Double deficiencies of Mst1 and Mst2 result in more severe impairment of lymphocyte trafficking and thymocyte egress with enhanced apoptosis [23] . Mst1-deficient T cells exhibit TCR-induced hyperproliferative responses [24] , but this phenotype was not confirmed with other gene-targeted mice [21] . Recently, mutations in STK4 / MST1 have been reported in patients with recurrent infections and autoimmune manifestations with autoantibodies, increased effector–memory subsets and hypergammaglobulinemia G and A [25] , [26] . The patients exhibited a progressive loss of naive CD4 + T cells, perhaps due to stress-induced apoptosis during severe infections [22] . Here we used thymic tissues to show that Mst1 −/− thymocytes are defective in LFA-1/ICAM-1-dependent high-velocity medullary migration. Mst1 is also required for migrating thymocytes to associate with rare populations of Aire + ICAM-1 hi mTECs in a negatively selecting environment. Consistent with this, thymocyte selection is impaired in Mst1 −/− mice, which develop T-cell-dependent autoimmunity with age. Our results suggest that Mst1 has a key role in regulating thymocyte self-antigen scanning in the medulla. Reduced migration velocities of Mst1 −/− SP thymocytes As Mst1 regulates lymphocyte trafficking in peripheral lymph nodes, we hypothesize that Mst1 is involved in scanning self-antigens by migrating thymocytes [27] . To explore this possibility, we used the thymic slice system into which purified thymocyte subsets were introduced and then measured the motility within thymic tissues by time-lapse imaging with a two-photon microscope [9] , [11] . Sorted DP cells and CD4 + SP cells ( Supplementary Fig. S1a ) from C57BL/6 and Mst1 −/− mice were introduced into thymic slices derived from CFP-transgenic mice to distinguish the cortex and medulla [11] . Consistent with previous work [11] , DP cells were exclusively localized in the cortex, whereas CD4 + SP cells predominantly migrated in the medulla ( Fig. 1a ; Supplementary Movies 1 and 2 ). The absence of Mst1 did not affect the localization of SP and DP cells ( Fig. 1b ). Wild-type and Mst1 −/− DP cells migrated similarly at ∼ 5.0 μm min −1 with no difference in displacement ( Fig. 1c ). DP cells express CD69 after interaction with positively selecting ligands. Wild-type CD69 + DP cells migrated slightly faster (6.7 mm min −1 ) than whole DP cells ( Fig. 1c ; Supplementary Fig. S2a ). The average speed of CD69 + Mst1 −/− DP cells were not significantly different ( P =0.19). In contrast, CD4 + SP cells migrated more rapidly in the cortex (14.3 μm min −1 ) and medulla (16.0 μm min −1 ). However, Mst1 −/− CD4 + SP cells greatly diminished velocities greater than 15 μm min −1 , resulting in reduced average velocities and the displacement ( Fig. 1d ). CD4 + SP cells contain newly generated (CD69 + ) and mature cells (CD69 − ) ( Supplementary Fig. S1 ). Mst1 deficiency decreased the average velocity of both CD69 + and CD69 − CD4SP cells ( Supplementary Fig. S2 ). These trafficking defects were not due to altered expression of CCR7 and LFA-1 ( Supplementary Fig. S3 ). 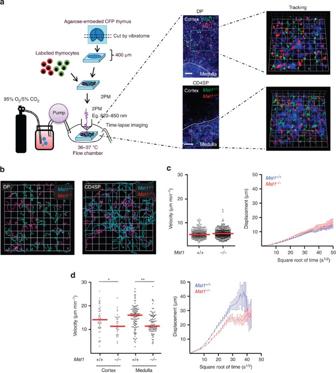Figure 1: Mst1 deficiency causes impaired migration of SP thymocytes within thymic tissues. (a) The experimental design used to analyse thymocyte migration in sliced thymic tissues using a two-photon microscope. CFSE (Mst1+/+) or CMTMR (Mst1−/−)-labelled DP or SP cells were cultured on the thymic slice for several hours, and then the thymocytes within the thymic slice were observed using a two-photon microscope. The thymic structures were visualized using ECFP mice. Individual images of slices with DP or SP cells illustrate the distinct migration patterns in the cortex and medulla (scale bar, 50 μm). The movements of individual cells were tracked. (b) The trajectories ofMst1+/+(sky blue) andMst1−/−(purple) DP or CD4SP cells are shown. (c) The average migration speed ofMst1+/+andMst1−/−DP in the cortex are shown in left panel. Bars indicate the median. Average displacements (±s.e.m.) from the origin plotted as a function of the square root of time are also shown in right panel. (d) The average migration speed ofMst1+/+andMst1−/−CD4SP cells in the cortex and medulla are shown. Bars indicate the median. Average displacements (±s.e.m.) from the origin plotted as a function of the square root of time are also shown. The raw tracking data for DP thymocytes (Mst1+/+,n=392;Mst1−/−,n=343) and the raw data for SP thymocytes (Mst1+/+, cortexn=49, medullan=123;Mst1−/−, cortexn=35, medullan=100) are from two independent experiments.Pvalues were calculated by Mann−WhitneyU-test, *0.01<P<0.05; **P<0.01. Figure 1: Mst1 deficiency causes impaired migration of SP thymocytes within thymic tissues. ( a ) The experimental design used to analyse thymocyte migration in sliced thymic tissues using a two-photon microscope. CFSE ( Mst1 +/+ ) or CMTMR ( Mst1 −/− )-labelled DP or SP cells were cultured on the thymic slice for several hours, and then the thymocytes within the thymic slice were observed using a two-photon microscope. The thymic structures were visualized using ECFP mice. Individual images of slices with DP or SP cells illustrate the distinct migration patterns in the cortex and medulla (scale bar, 50 μm). The movements of individual cells were tracked. ( b ) The trajectories of Mst1 +/+ (sky blue) and Mst1 −/− (purple) DP or CD4SP cells are shown. ( c ) The average migration speed of Mst1 +/+ and Mst1 −/− DP in the cortex are shown in left panel. Bars indicate the median. Average displacements (±s.e.m.) from the origin plotted as a function of the square root of time are also shown in right panel. ( d ) The average migration speed of Mst1 +/+ and Mst1 −/− CD4SP cells in the cortex and medulla are shown. Bars indicate the median. Average displacements (±s.e.m.) from the origin plotted as a function of the square root of time are also shown. The raw tracking data for DP thymocytes ( Mst1 +/+ , n =392; Mst1 −/− , n =343) and the raw data for SP thymocytes ( Mst1 +/+ , cortex n =49, medulla n =123; Mst1 −/− , cortex n =35, medulla n =100) are from two independent experiments. P values were calculated by Mann−Whitney U -test, *0.01< P <0.05; ** P <0.01. Full size image Rapid SP thymocyte migration mediated by LFA-1 and ICAM-1 As Mst1 regulates LFA-1 (ref. 20 ), we speculated that integrin-dependent processes may be involved in SP thymocyte trafficking in the medulla. In support of this possibility, ICAM-1 was expressed throughout the thymic tissue with greater expression in the medulla than the cortex ( Fig. 2a ). ICAM-1 was expressed in CD11c + DCs and mTECs ( Fig. 2b ). Interestingly, high-density ICAM-1 foci were scattered throughout the medulla. The high-density ICAM-1 was associated with Aire + mTECs, but not CD11c + DCs ( Fig. 2c ). ICAM-1 immunostaining was completely abolished in an ICAM-1 −/− thymus, confirming the specificity of the antibody ( Fig. 2d ). 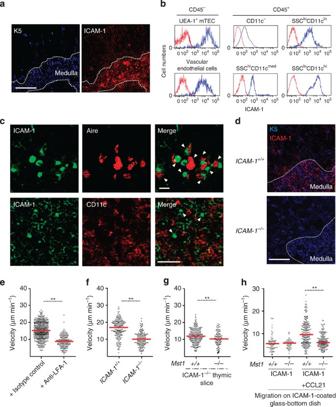Figure 2: Requirement of LFA-1and ICAM-1 for efficient migration in thymic tissues. (a) Immunostaining of ICAM-1 and keratin5 (K5) of the thymus. Scale bar, 100 μm. (b) The levels of ICAM-1 expression in CD45−UEA-1+mTECs and CD45−CD31+vascular endothelial cells, CD45+CD11c−and CD11c-low and high expressing cells. (c) Co-staining for ICAM-1 and Aire (upper panels, scale bar, 10 μm) or CD11c (lower panels, scale bar, 50 μm). Arrowheads indicate ICAM-1 bright foci. Note the close association of Aire in nuclei and ICAM-1 foci. (d) Immunostaining of theICAM-1+/+andICAM-1−/−thymus with anti-ICAM-1 (red) and anti-keratin 5 antibodies (blue). Scale bar, 100 μm. (e) The average velocity of CD4+SP cells in the thymic medulla in the absence or presence of an anti-LFA-1 antibody (KBA) is shown (+isotype control,n=513; +anti-LFA-1,n=171 from two independent experiments). (f) The average velocity of CD4+SP cells in the medulla ofICAM-1+/+orICAM-1−/−thymic tissues is also shown (ICAM-1+/+slice,n=190;ICAM-1−/−slice,n=148 from two independent experiments). (g) The migration speed ofMst1−/−CD4SP cells withinICAM-1−/−thymic tissues (Mst1+/+slice,n=226;Mst1−/−slice,n=103). (h) The migration velocities ofMst1+/+andMst1−/−CD4+SP cells on ICAM-1-coated substrates.Mst1+/+andMst1−/−CD4+SP cells were differentially labelled and incubated on the ICAM-1-coated surface (0.8 μg ml−1) with or without immobilized CCL21. The average velocity of CD4+SP cells from three independent experiments is shown (ICAM-1,Mst1+/+,n=78,Mst1−/−,n=59; ICAM-1+ CCL21,Mst1+/+,n=214,Mst1−/−, n=176). Bars indicate the median.P-values were calculated by Mann−WhitneyU-test ***P<0.01. Figure 2: Requirement of LFA-1and ICAM-1 for efficient migration in thymic tissues. ( a ) Immunostaining of ICAM-1 and keratin5 (K5) of the thymus. Scale bar, 100 μm. ( b ) The levels of ICAM-1 expression in CD45 − UEA-1 + mTECs and CD45 − CD31 + vascular endothelial cells, CD45 + CD11c − and CD11c-low and high expressing cells. ( c ) Co-staining for ICAM-1 and Aire (upper panels, scale bar, 10 μm) or CD11c (lower panels, scale bar, 50 μm). Arrowheads indicate ICAM-1 bright foci. Note the close association of Aire in nuclei and ICAM-1 foci. ( d ) Immunostaining of the ICAM-1 +/+ and ICAM-1 −/− thymus with anti-ICAM-1 (red) and anti-keratin 5 antibodies (blue). Scale bar, 100 μm. ( e ) The average velocity of CD4 + SP cells in the thymic medulla in the absence or presence of an anti-LFA-1 antibody (KBA) is shown (+isotype control, n =513; +anti-LFA-1, n =171 from two independent experiments). ( f ) The average velocity of CD4 + SP cells in the medulla of ICAM-1 +/+ or ICAM-1 −/− thymic tissues is also shown ( ICAM-1 +/+ slice, n =190; ICAM-1 −/− slice, n =148 from two independent experiments). ( g ) The migration speed of Mst1 −/− CD4SP cells within ICAM-1 −/− thymic tissues ( Mst1 +/+ slice, n =226; Mst1 −/− slice, n =103). ( h ) The migration velocities of Mst1 +/+ and Mst1 −/− CD4 + SP cells on ICAM-1-coated substrates. Mst1 +/+ and Mst1 −/− CD4 + SP cells were differentially labelled and incubated on the ICAM-1-coated surface (0.8 μg ml −1 ) with or without immobilized CCL21. The average velocity of CD4 + SP cells from three independent experiments is shown (ICAM-1, Mst1 +/+ , n =78, Mst1 −/− , n =59; ICAM-1+ CCL21, Mst1 +/+ , n =214, Mst1 −/− , n =176). Bars indicate the median. P -values were calculated by Mann−Whitney U -test *** P <0.01. Full size image To examine the requirement of LFA-1 and ICAM-1 in thymocyte migration, we monitored the migration of CD4 + SP cells in thymic tissues with or without an anti-LFA-1 antibody (KBA) [28] . Compared with the isotype control antibody, the anti-LFA antibody decreased the instantaneous velocities of CD4 + SP cells in the medulla by 43% compared with the control (8.8 versus 15.2 μm min −1 ; Fig. 2e ; Supplementary Movie 3 ). A similar reduction was also observed in thymic slices from ICAM-1 −/− mice (9.9 versus 16.9 μm min −1 ; Fig. 2f ; Supplementary Movie 4 ). These results indicate that LFA-1 and ICAM-1 are required for the high-velocity migration of SP cells in the medulla. To examine the role of Mst1 in CD4 + SP cell migration within ICAM-1-deficient tissues, we compared the migration of Mst1 +/+ and Mst1 −/− CD4 + SP cells in ICAM-1-deficient thymic tissues. There was a mild, but significant decrease of velocities of Mst1 −/− cells ( P =0.001; Fig 2g ), suggesting an involvement of other medullary substrates or integrin-independent mechanisms. To directly confirm whether SP cells can migrate on ICAM-1, CD4 + SP cells from wild-type and Mst1 −/− mice were monitored on an ICAM-1-coated surface ( Fig. 2h ; Supplementary Movie 5 ). With ICAM-1 alone, the majority of the CD4 + SP cells were sessile with a minor population exhibiting active migration, which was rarely observed with Mst1 −/− CD4 + SP cells. The medullary chemokine CCL21 stimulated CD4 + SP cell motility on ICAM-1, showing an average velocity of 9.6 μm min −1 and a maximum speed greater than 20 μm min −1 . In contrast, Mst1 −/− CD4 + SP cells showed a limited response to CCL21 with average 6.0 μm min −1 ( Fig. 2h ). These results indicate that Mst1 is required for high-velocity medullary migration of CD4 + SP cells via LFA-1 and ICAM-1. DP thymocytes failed to migrate on ICAM-1 even in the presence of CXCL12 (data not shown), which is consistent with the inability of DP cells to enter and migrate in an ICAM-1-rich medulla. Antigen-specific association of SP cells with mTECs To investigate how medullary SP thymocytes interact with antigen-presenting cells (APCs) expressing self-antigen, we used the Aire-dependent negative selection system to conduct two-photon imaging of thymocytes in an environment expressing a negatively selecting ligand [6] . In this system, mTECs express membrane-bound ovalbumin under the control of the rat insulin promoter and induce the deletion of OT-II SP thymocytes in an Aire-dependent manner [29] , [30] . Thymic slices were prepared from wild-type C57BL/6 and RIP-mOVA transgenic mice into which purified polyclonal wild-type and OT-II CD4 + SP ( Supplementary Fig. S1 ) were simultaneously introduced. After 5 h, live imaging of the thymic slices showed that both wild-type and OT-II CD4 + SP cells migrated vigorously within wild-type thymic tissues with comparable velocities ( Fig. 3a and Supplementary Movie 6 , data not shown). However, in the RIP-mOVA tissues, the introduced SP cells formed cell clusters, which were composed exclusively of OT-II CD4 + SP cells, whereas wild-type CD4 + SP cells were rarely involved in these clusters ( Fig. 3a and Supplemental Movie 6 ). These results indicate that OT-II CD4 + SP cells form antigen-dependent clusters. Consistent with this finding, high intracellular calcium levels were detected in clustered CD4 + SP cells, which contrasted the relatively low calcium levels in migrating OT-II CD4 + SP cells with or without the negatively selecting ligand, indicating that signalling occurred through antigen-engaged TCRs ( Fig. 3b ). To clarify the cell dynamics of OT-II CD4 + SP cells in the presence of the negatively selecting ligand, CD4 + SP cells were monitored in RIP-mOVA tissues at 1, 5 and 24 h after cell loading. Within 1 h, ∼ 40% of OT-II CD4 + SP cells were quickly arrested in the medullary region, resulting in an increase in populations with velocities <5 μm min −1 ( Fig. 3c ). By 5 h, OT-II CD4 + SP cells formed clusters with average velocities <5 μm min −1 , whereas other migrating CD4 + SP exhibited velocities of ∼ 12 μm min −1 , which was lower than the average speed of polyclonal thymocytes (15−16 μm min −1 ). At 24 h, these clusters were dissociated with a reciprocal increase in CD4 + SP cell velocities ( Fig. 3c ). 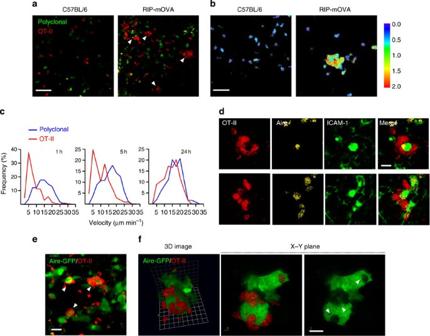Figure 3: Antigen-specific thymocyte cluster formation in the thymic medulla of RIP-mOVA mice. (a) OT-II CD4+SP cells (red) and polyclonal CD4+SP cells (green) in thymic tissues derived from C57BL/6 (left) and RIP-mOVA transgenic mice (right). Representative images at 5 h after cell loading are shown. Note that cell cluster formation of OT-II CD4+SP cells in RIP-mOVA tissues (arrowheads). Scale bar, 40 μm. Time-lapse recordings are inSupplementary Movie 6. (b) The intracellular calcium concentration in OT-II CD4+SP cells in C57BL/6- (left) or RIP-mOVA transgenic (right)-derived thymic slices was measured based on the ratiometric calcium indicator Indo-PE3. The calcium concentration was visualized based on the ratio of bound/unbound Ca2+, as shown in the hue graph. Scale bar, 25 μm. (c) The migration velocity dynamics of polyclonal C57BL/6 CD4+SP cells (blue) and OT-II CD4+SP cells (red) in RIP-mOVA transgenic-derived thymic tissues measured at 1, 5 and 24 h after cell loading. (d) Cells associated with OT-II SP cell clusters were visualized by immunostaining frozen sections with anti-ICAM-1 and anti-Aire antibodies. Note that OT-II CD4+SP cell clusters were associated with Aire+ICAM-1hicells. Scale bar, 10 μm. (e) Cluster formation of OT-II CD4+SP cells (red) with Aire-GFP+cells (green) in an RIP-mOVA transgenic/Aire-GFP+/−knock-in thymic slice. Scale bar, 20 μm. Time-lapse recordings are inSupplementary Movie 7. (f) Enlarged 3D andx–yplane views of clusters of OT-II CD4+SP cells (red) with Aire-GFP+cells as ine. Note that some OT-II CD4+SP cells are inside Aire-GFP+cells (arrowheads), as indicated by sharp boundaries of GFP-negative regions of the cell body in thex–yfocal plane (views with or without display of OT-II CD4+SP). Scale bar, 10 μm. Figure 3: Antigen-specific thymocyte cluster formation in the thymic medulla of RIP-mOVA mice. ( a ) OT-II CD4 + SP cells (red) and polyclonal CD4 + SP cells (green) in thymic tissues derived from C57BL/6 (left) and RIP-mOVA transgenic mice (right). Representative images at 5 h after cell loading are shown. Note that cell cluster formation of OT-II CD4 + SP cells in RIP-mOVA tissues (arrowheads). Scale bar, 40 μm. Time-lapse recordings are in Supplementary Movie 6 . ( b ) The intracellular calcium concentration in OT-II CD4 + SP cells in C57BL/6- (left) or RIP-mOVA transgenic (right)-derived thymic slices was measured based on the ratiometric calcium indicator Indo-PE3. The calcium concentration was visualized based on the ratio of bound/unbound Ca 2+ , as shown in the hue graph. Scale bar, 25 μm. ( c ) The migration velocity dynamics of polyclonal C57BL/6 CD4 + SP cells (blue) and OT-II CD4 + SP cells (red) in RIP-mOVA transgenic-derived thymic tissues measured at 1, 5 and 24 h after cell loading. ( d ) Cells associated with OT-II SP cell clusters were visualized by immunostaining frozen sections with anti-ICAM-1 and anti-Aire antibodies. Note that OT-II CD4 + SP cell clusters were associated with Aire + ICAM-1 hi cells. Scale bar, 10 μm. ( e ) Cluster formation of OT-II CD4 + SP cells (red) with Aire-GFP + cells (green) in an RIP-mOVA transgenic/Aire-GFP +/− knock-in thymic slice. Scale bar, 20 μm. Time-lapse recordings are in Supplementary Movie 7 . ( f ) Enlarged 3D and x – y plane views of clusters of OT-II CD4 + SP cells (red) with Aire-GFP + cells as in e . Note that some OT-II CD4 + SP cells are inside Aire-GFP + cells (arrowheads), as indicated by sharp boundaries of GFP-negative regions of the cell body in the x – y focal plane (views with or without display of OT-II CD4 + SP). Scale bar, 10 μm. Full size image To identify the APC that supports cluster formation, frozen sections of thymic slice cultures in the above experiment were immunostained. We found that OT-II SP cells frequently associated with Aire + ICAM-1 hi mTECs, in which cells were located in close apposition to high-density ICAM-1 ( Fig. 3d ). More than 70% OT-II SP cells (41 Aire + clusters out of 53 clusters) were in contact with Aire + cells. To demonstrate the direct association with Aire + mTECs, thymic slices from Aire-GFP knock-in mice expressing RIP-mOVA were used for live imaging ( Fig. 3e ). Actively migrating OT-II CD4 + SP cells arrested and were associated directly with GFP + mTECs ( Fig. 3e and Supplementary Movie 7 ). Interestingly, some CD4 + SP cells penetrated into the cell body of Aire-GFP + mTECs ( Fig. 3f ). In contrast, apparent cluster formations of OT-II CD4 + SP cells with CD11c + DCs were not detected by immunostaining or using thymic slices from CD11c-YFP transgenic mice (data not shown). Few dying cells were detected within an imaging time ( ∼ 24 h; Supplementary Fig. S4 ), as is the case using the OT-I/RIP-mOVA system [10] , suggesting that negative selection takes a longer time beyond 24 h. OT-II SP cells dissociated from mTEC would be dying during subsequent migration and brief contacts with surrounding dendritic cells [10] . Impaired associations of Mst1 −/− SP thymocytes with mTECs We then examined the effects of the absence of Mst1 on the ability of OT-II CD4 + SP cells to form clusters with mTECs. When introduced into RIP-mOVA thymic slices, Mst1 −/− OT-II SP cells exhibited reduced arrest frequencies and cluster formation with an increase in slowly migrating cells (5−10 μm min −1 ; Fig. 4a ; Supplementary Movie 8 ). The cluster numbers of Mst1 −/− OT-II SP thymocytes were reduced by approximately half ( Fig. 4b , P =0.01). To compare cluster formation between wild-type and Mst1 −/− OT-II SP cells in the same environment, we simultaneously introduced wild-type and Mst1 −/− OT-II CD4 + SP thymocytes into the same RIP-mOVA thymic tissue ( Fig. 4c ). After 5–9 h, the ratio of Mst1 −/− OT-II SP cells to wild-type SP cells was 0.57, which was significantly lower than the ratio of differentially labelled wild-type cells in the clusters (1.0, P =0.002; Fig. 4c ). The inefficient cluster formations by Mst1 deficiency were also observed in CD69 + CD4 + SP cells ( Fig. 4d ). 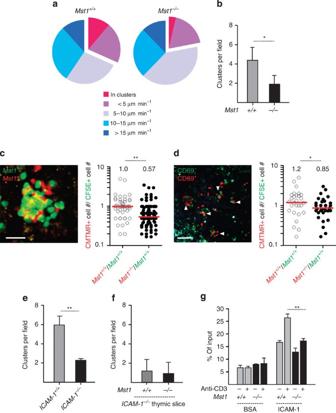Figure 4: Mst1 deficiency results in inefficient cluster formation. (a) Profiles of the migration velocities of OT-IIMst1+/+andMst1−/−CD4+SP cells in RIP-mOVA thymic tissues 5 h after cell loading (5×104each). (b) Cluster formation byMst1+/+andMst1−/−OT-II CD4+SP cells (1×105each) was quantified throughout the thymic tissues derived from RIP transgenic mice. The cluster numbers per field (right,xyz, 340×340×100 μm3) are shown. The data are representative of two independent experiments. (c) Representative images of the cluster (left) and ratios (right) ofMst1+/+OT-II SP cells (green) andMst1−/−OT-II SP cells (red) in clusters within the RIP-mOVA thymic tissues (scale bar, 20 μm). The ratios of differentially labelledMst1+/+OT-II SP cells and the ratio of differentially labelledMst1+/+andMst1−/−OT-II SP cells in a single cluster (Mst1+/+/Mst1+/+,n=49;Mst1−/−/Mst1+/+,n=93 from two or three independent experiments) are shown. (d) A representative image 5 h after cell loading of CD69+OT-II SP (red) and CD69−OT-II SP (green) in thymic tissues derived from RIP-mOVA transgenic mice is shown (scale bar, 50 μm). Arrowhead indicates clusters formed by CD69+and CD69−OT-II SP cells. The ratios of differentially labelledMst1+/+OT-II SP cells and the ratio of differentially labelledMst1+/+andMst1−/−OT-II SP cells in a single cluster are shown in the right panel (Mst1+/+/Mst1+/+,n=28;Mst1−/−/Mst1+/+,n=34). (e) Impaired cluster formation of OT-II SP cells inICAM-1−/−thymic slices. Cluster numbers per field (xyz, 340×340×100 μm3) by OT-II SP cells inICAM-1+/+orICAM-1−/−thymic tissues at 8–9 h were counted using a two-photon microscope. (f) Cluster formations ofMst1−/−andMst1+/+OT-II SP cells inICAM-1−/−thymic slices. (g) Adhesion ofMst1+/+andMst1−/−CD4 SP cells to ICAM-1 and BSA with and without anti-CD3 antibody are measured in triplicates and expressed as a percentage of bound cells to input cells. The average±s.d. are shown.Pvalues were calculated by Mann–WhitneyU-test (d–f) or unpaired Student'st-test (g); *0.01<P<0.05; **P<0.01. Figure 4: Mst1 deficiency results in inefficient cluster formation. ( a ) Profiles of the migration velocities of OT-II Mst1 +/+ and Mst1 −/− CD4 + SP cells in RIP-mOVA thymic tissues 5 h after cell loading (5×10 4 each). ( b ) Cluster formation by Mst1 +/+ and Mst1 −/− OT-II CD4 + SP cells (1×10 5 each) was quantified throughout the thymic tissues derived from RIP transgenic mice. The cluster numbers per field (right, xyz , 340×340×100 μm 3 ) are shown. The data are representative of two independent experiments. ( c ) Representative images of the cluster (left) and ratios (right) of Mst1 +/+ OT-II SP cells (green) and Mst1 −/− OT-II SP cells (red) in clusters within the RIP-mOVA thymic tissues (scale bar, 20 μm). The ratios of differentially labelled Mst1 +/+ OT-II SP cells and the ratio of differentially labelled Mst1 +/+ and Mst1 −/− OT-II SP cells in a single cluster ( Mst1 +/+ /Mst1 +/+ , n =49; Mst1 −/− /Mst1 +/+ , n =93 from two or three independent experiments) are shown. ( d ) A representative image 5 h after cell loading of CD69 + OT-II SP (red) and CD69 − OT-II SP (green) in thymic tissues derived from RIP-mOVA transgenic mice is shown (scale bar, 50 μm). Arrowhead indicates clusters formed by CD69 + and CD69 − OT-II SP cells. The ratios of differentially labelled Mst1 +/+ OT-II SP cells and the ratio of differentially labelled Mst1 +/+ and Mst1 −/− OT-II SP cells in a single cluster are shown in the right panel ( Mst1 +/+ /Mst1 +/+ , n =28; Mst1 −/− /Mst1 +/+ , n =34). ( e ) Impaired cluster formation of OT-II SP cells in ICAM-1 −/− thymic slices. Cluster numbers per field ( xyz , 340×340×100 μm 3 ) by OT-II SP cells in ICAM-1 +/+ or ICAM-1 −/− thymic tissues at 8–9 h were counted using a two-photon microscope. ( f ) Cluster formations of Mst1 −/− and Mst1 +/+ OT-II SP cells in ICAM-1 −/− thymic slices. ( g ) Adhesion of Mst1 +/+ and Mst1 −/− CD4 SP cells to ICAM-1 and BSA with and without anti-CD3 antibody are measured in triplicates and expressed as a percentage of bound cells to input cells. The average±s.d. are shown. P values were calculated by Mann–Whitney U -test ( d – f ) or unpaired Student's t -test ( g ); *0.01< P <0.05; ** P <0.01. Full size image To determine whether the interactions of SP thymocytes with mTECs require LFA-1 and ICAM-1, we measured cluster formation of OT-II CD4 + SP cells within ICAM-1 −/− RIP-mOVA thymic tissues. Cluster formation was significantly decreased in ICAM-1 −/− tissues ( Fig. 4e ; Supplementary Movie 9 ). We also examine the cluster formation of wild-type and Mst1 −/− CD4 + SP cells within ICAM-1 −/− RIP-mOVA thymic slice. There were little synergistic effects on cluster formations with mTEC ( Fig. 4f ), suggesting that Mst1 is required for ICAM-1-dependent cluster formation with antigen-presenting mTEC. Consistently, Mst1 −/− CD4 + SP cells exhibited impaired TCR-induced adhesion to ICAM-1 in vitro ( Fig. 4g ). Thus, these results suggest that Mst1 is required for efficient scanning with self-antigen presenting Aire + mTECs through ICAM-1. Reduced positive selection of Mst1 −/− thymocytes To explore a possibility that Mst1 deficiency might affect thymocyte selection, we used MHC class I-restricted male H-Y antigen-specific TCR transgenic mice in which CD8 + SP cells are positively selected. We found that the percentage of CD8 + SP cells in female H-Y TCR transgenic mice was reduced from 25.4 to 9.2% ( Fig. 5a ). When the newly selected CD69 hi SP subset in those mice was measured, both the CD69 hi T3.70 + CD8 + SP cell percentage and numbers in Mst1 −/− H-Y TCR transgenic mice were severely decreased by 70% ( P =0.0002 and P =0.016), compared with Mst1 +/+ H-Y mice ( Fig. 5b ). We also confirmed the defect in positive selection because of the Mst1 deficiency by bone marrow (BM) chimera. A comparison of the CD69 + TCRβ + CD4 + SP or CD8 + SP subset within the Mst1 +/+ and Mst1 −/− population showed that there were significant reductions by 30% ( P =0.007) and 63% ( P =0.0004), respectively ( Fig. 5c,d ). The Mst1 −/− (CD45.2) population in the thymus was reduced to ∼ 10% compared with the Mst1 +/+ population (CD45.1), suggesting that the homing of T-cell progenitors to the thymus was impaired ( Fig. 5c ). Reduced positive selection was not due to an inefficient reconstitution from Mst1 −/− donor cells, as there were no differences in the CD69 + TCRβ + CD8 + SP subsets between Mst1 +/+ CD45.1 and Mst1 +/+ CD45.2 donor cells when mixed at a 9:1 reconstitution ratio ( Fig. 5e ). These results indicate that defective positive selection in the Mst1 −/− thymus is intrinsic to thymocytes. Of note, CD69 + TCR + DP cells were not altered in either transgenic or chimeric mice ( Fig. 5f,g ), suggesting that the defect in positive selection occurred at the transition from the CD69 + DP to SP stage. 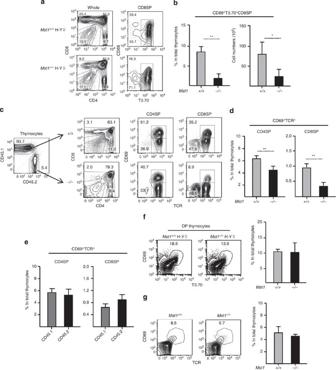Figure 5: Mst1 deficiency results in impaired generation of SP thymocytes. (a) The expression levels of CD4 and CD8 on total thymocytes and CD69 and T3.70 (clonotypic TCR) on CD8+SP thymocytes from H-Y TCR+Mst1+/+mice (n=4) and H-Y TCR+Mst1−/−mice (n=4) are shown. The numbers in the quadrants indicate the percent of cells in the gate. (b) The bar graphs show the percentage (left panel) and cell numbers (right panel) of CD69+T3.70 among the total thymocytes. (c) CD45.1 and CD45.2 expression and thymocyte subsets in mice reconstituted with a mixture ofMst1+/+(CD45.1+) andMst1−/−(CD45.2+) BM cells (n=4). (d) The graphs show the percentage of CD69+CD4+SP cells (left panel) and CD69+CD8+SP cells (right panel) among CD45.1+thymocytes or CD45.2+thymocytes of chimeric mice. The bar in the graphs indicates the average±s.d. (e) Equivalent reconstitution ofMst1+/+CD45.1+andMst1+/+CD45.2+BM cells. Mice were reconstituted with a mixture at a 9:1 reconstitution ratio ofMst1+/+(CD45.1+) andMst1+/+(CD45.2+) BM cells (n=3). The percentage of CD69+CD4+SP cells and CD69+CD8+SP cells among CD45.1+thymocytes or CD45.2+thymocytes in the chimeric mice. The bar in the graphs indicates the average±s.d. (f) Intact CD69+TCR+DP thymocytes inMst1−/−mice. Expression of CD69 and T3.70 (clonotypic TCR) on DP thymocytes from H-Y TCR+Mst1+/+(n=4) and H-Y TCR+Mst1−/−mice (n=4) are shown. The numbers indicate the percent of cells in the gate. The bar graphs show the percentage of CD69+T3.70 DP cells among the total thymocytes of those mice. (g) CD69 and TCRβ expression on DP cells in the thymus of mice reconstituted with a mixture ofMst1+/+(CD45.1) andMst1−/−(CD45.2) BM cells (n=4). The bar graph shows the percentage of CD69+DP cells among CD45.1+thymocytes or CD45.2+thymocytes of the chimeric mice. The bar in the graphs indicates the average±s.d.Pvalues were calculated by unpaired (b,d,f) or paired (d,e,g) Student'st-test; *0.01<P<0.05; **P<0.01. Figure 5: Mst1 deficiency results in impaired generation of SP thymocytes. ( a ) The expression levels of CD4 and CD8 on total thymocytes and CD69 and T3.70 (clonotypic TCR) on CD8 + SP thymocytes from H-Y TCR + Mst1 +/+ mice ( n =4) and H-Y TCR + Mst1 −/− mice ( n =4) are shown. The numbers in the quadrants indicate the percent of cells in the gate. ( b ) The bar graphs show the percentage (left panel) and cell numbers (right panel) of CD69 + T3.70 among the total thymocytes. ( c ) CD45.1 and CD45.2 expression and thymocyte subsets in mice reconstituted with a mixture of Mst1 +/+ (CD45.1 + ) and Mst1 −/− (CD45.2 + ) BM cells ( n =4). ( d ) The graphs show the percentage of CD69 + CD4 + SP cells (left panel) and CD69 + CD8 + SP cells (right panel) among CD45.1 + thymocytes or CD45.2 + thymocytes of chimeric mice. The bar in the graphs indicates the average±s.d. ( e ) Equivalent reconstitution of Mst1 +/+ CD45.1 + and Mst1 +/+ CD45.2 + BM cells. Mice were reconstituted with a mixture at a 9:1 reconstitution ratio of Mst1 +/+ (CD45.1 + ) and Mst1 +/+ (CD45.2 + ) BM cells ( n =3). The percentage of CD69 + CD4 + SP cells and CD69 + CD8 + SP cells among CD45.1 + thymocytes or CD45.2 + thymocytes in the chimeric mice. The bar in the graphs indicates the average±s.d. ( f ) Intact CD69 + TCR + DP thymocytes in Mst1 −/− mice. Expression of CD69 and T3.70 (clonotypic TCR) on DP thymocytes from H-Y TCR + Mst1 +/+ ( n =4) and H-Y TCR + Mst1 −/− mice ( n =4) are shown. The numbers indicate the percent of cells in the gate. The bar graphs show the percentage of CD69 + T3.70 DP cells among the total thymocytes of those mice. ( g ) CD69 and TCRβ expression on DP cells in the thymus of mice reconstituted with a mixture of Mst1 +/+ (CD45.1) and Mst1 −/− (CD45.2) BM cells ( n =4). The bar graph shows the percentage of CD69 + DP cells among CD45.1 + thymocytes or CD45.2 + thymocytes of the chimeric mice. The bar in the graphs indicates the average±s.d. P values were calculated by unpaired ( b , d , f ) or paired ( d , e , g ) Student's t -test; *0.01< P <0.05; ** P <0.01. Full size image Negative selection in Mst1 −/− mice To determine whether Mst1 deficiency alters negative selection against self-antigen, we first examined male H-Y TCR transgenic mice. In male H-Y transgenic mice, immature thymocytes were deleted from the DP stage [31] . In male H-Y Mst1 −/− mice, DP thymocytes tended to be increased, although this increase was not statistically significant ( P =0.25; Fig. 6a,b ). As H-Y male antigen is broadly expressed with deletion occurring in the early developmental stage of thymocytes, we examined negative selection against organ-specific antigen in the medulla using the RIP-mOVA-OT-II system. We reconstituted RIP-mOVA mice with a mixture of equal numbers of Mst1 +/+ OT-II (CD45.1 + CD45.2 + ) and Mst1 −/− OT-II (CD45.2) BM cells. After 5–8 weeks, we measured the deletion of the most mature HSA lo V β 5 + CD4 + SP cells [29] in CD45.1 + CD45.2 + or CD45.2 + thymocytes ( Fig. 6c–f ). Mature HSA lo V β 5 + CD4 + SP cells were increased twice in Mst1 −/− OT-II cells compared with Mst1 +/+ OT-II cells ( Fig. 6c ), consistent with impaired thymocyte egress. The deletion of HSA lo V β 5 Mst1 −/− OT-II cells in RIP-mOVA mice was inefficient ( Fig. 6c,d ), as Mst1 −/− HSA lo V β 5 + CD4 + SP thymocytes was increased approximately threefold, compared with Mst1 +/+ CD4 + SP thymocytes ( P =0.024; Fig. 6d ). Thymic negative selection of OT-II thymocytes results in a decreased number of peripheral OT-II cells. Consistently, the reduction in the percentage of Vα2 + Vβ5 + cells in Mst1 −/− CD45.1 − CD4 + T cells was less efficient compared with wild-type cells ( Fig. 6e,f ). Taken together, these results suggest that Mst1 −/− thymocytes have an intrinsic impairment in tissue-specific antigen recognition in addition to thymocyte egress. 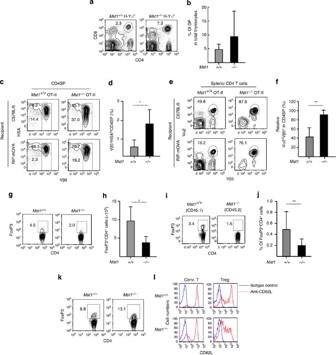Figure 6: Mst1 deficiency impairs negative selection of SP thymocytes and thymic Treg generation. (a) Negative selection in the thymus ofMst1−/−H-Y TCR transgenic mice. Flow cytometric profiles of CD4 and CD8 expression among thymocytes. (b) Percentages (average±s.d.) of DP thymocytes inMst1+/+andMst1−/−H-Y TCR transgenic mice (P=0.25). (c) Experiments from C57BL/6 (n=4) or RIP-mOVA transgenic (n=5) mice (CD45.1+CD45.2+) reconstituted with a mixture ofMst1+/+(CD45.1+CD45.2+) andMst1−/−(CD45.2+) OT-II transgenic BM cells are shown. Representative FACS profiles of HSAhiVβ5+and HSAloVβ5+onMst1+/+orMst1−/−CD4+SP cells in the BM chimeric mice. The numbers in the quadrants indicate the percent of cells in the gate. (d) The percentages ofMst1+/+orMst1−/−HSAloVβ5+CD4+SP cells in RIP-mOVA recipients. (e) Vα2 and Vβ5 expression onMst1+/+orMst1−/−splenic CD4+T cells. (f) The relative percentages of Vα2+Vβ5+inMst1+/+orMst1−/−CD4+splenic T cells compared with controls. (g) The percentage of FoxP3+CD4+inMst1+/+andMst1−/−thymocytes. (h) Numbers of FoxP3+CD4+cells inMst1+/+andMst1−/−thymocytes. (i) The reduction in FoxP3+CD4+cells is intrinsic to thymocytes. The flow cytometric profiles of FoxP3 expression in CD4+SP cells from mice reconstituted with a mixture ofMst1+/+(CD45.1+) andMst1−/−(CD45.2+) BM cells (n=4). (j) The percentage of FoxP3+CD4+cells inMst1+/+thymocytes or that ofMst1−/−thymocytes in chimeric mice. The bar in the graphs indicates the average (±s.d.). (k) FoxP3+regulatory T cells in the periphery ofMst1−/−mice. Expression of FoxP3 in CD4+splenic T cells fromMst1+/+andMst1−/−mice. (l) The CD62L expression levels in FoxP3−CD4+(Conv. T) and FoxP3+CD4+(Treg) inMst1+/+andMst1−/−mice are shown. The blue and red lines represent the staining intensity with the isotype control and anti-CD62L antibody, respectively.Pvalues were calculated by unpaired (b,h) or paired (d,f,j) Student'st-test, *0.01<P<0.05; **P<0.01. Figure 6: Mst1 deficiency impairs negative selection of SP thymocytes and thymic Treg generation. ( a ) Negative selection in the thymus of Mst1 −/− H-Y TCR transgenic mice. Flow cytometric profiles of CD4 and CD8 expression among thymocytes. ( b ) Percentages (average±s.d.) of DP thymocytes in Mst1 +/+ and Mst1 −/− H-Y TCR transgenic mice ( P =0.25). ( c ) Experiments from C57BL/6 ( n =4) or RIP-mOVA transgenic ( n =5) mice (CD45.1 + CD45.2 + ) reconstituted with a mixture of Mst1 +/+ (CD45.1 + CD45.2 + ) and Mst1 −/− (CD45.2 + ) OT-II transgenic BM cells are shown. Representative FACS profiles of HSA hi Vβ5 + and HSA lo Vβ5 + on Mst1 +/+ or Mst1 −/− CD4 + SP cells in the BM chimeric mice. The numbers in the quadrants indicate the percent of cells in the gate. ( d ) The percentages of Mst1 +/+ or Mst1 −/− HSA lo Vβ5 + CD4 + SP cells in RIP-mOVA recipients. ( e ) Vα2 and Vβ5 expression on Mst1 +/+ or Mst1 −/− splenic CD4 + T cells. ( f ) The relative percentages of Vα2 + Vβ5 + in Mst1 +/+ or Mst1 −/− CD4 + splenic T cells compared with controls. ( g ) The percentage of FoxP3 + CD4 + in Mst1 +/+ and Mst1 −/− thymocytes. ( h ) Numbers of FoxP3 + CD4 + cells in Mst1 +/+ and Mst1 −/− thymocytes. ( i ) The reduction in FoxP3 + CD4 + cells is intrinsic to thymocytes. The flow cytometric profiles of FoxP3 expression in CD4 + SP cells from mice reconstituted with a mixture of Mst1 +/+ (CD45.1 + ) and Mst1 −/− (CD45.2 + ) BM cells ( n =4). ( j ) The percentage of FoxP3 + CD4 + cells in Mst1 +/+ thymocytes or that of Mst1 −/− thymocytes in chimeric mice. The bar in the graphs indicates the average (±s.d.). ( k ) FoxP3 + regulatory T cells in the periphery of Mst1 −/− mice. Expression of FoxP3 in CD4 + splenic T cells from Mst1 +/+ and Mst1 −/− mice. ( l ) The CD62L expression levels in FoxP3 − CD4 + (Conv. T) and FoxP3 + CD4 + (Treg) in Mst1 +/+ and Mst1 −/− mice are shown. The blue and red lines represent the staining intensity with the isotype control and anti-CD62L antibody, respectively. P values were calculated by unpaired ( b , h ) or paired ( d , f , j ) Student's t -test, *0.01< P <0.05; ** P <0.01. Full size image Defective regulatory T-cell development in Mst1 −/− mice Regulatory T cells (Tregs) develop through a selection process that involves strong signalling of a self-ligand in the thymus [32] , [33] . To examine Treg development, we measured the number of FoxP3 + CD4 + cells in the thymus of 2-month-old Mst1 −/− mice. Compared with controls, the number of FoxP3 + CD4 + Tregs were reduced by 60% ( Fig. 6g,h ). We confirmed the reduced Tregs in the thymus were intrinsic to thymocytes with mixed BM chimeric mice ( Fig. 6i,j ). Foxo1 and Foxo3 are required for proper Treg development in the thymus through regulation of Foxp3 promoter activity [34] . However, Mst1-deficient and wild-type thymocytes expressed Foxo1 and Foxo3 comparably ( Supplementary Fig. S5 ). In contrast, peripheral FoxP3 + CD62L lo -induced Tregs were recovered in Mst1 −/− mice ( Fig. 6k,l ). We did not detect a significant difference in CTLA-4 expression or in the suppressive functions on the proliferation of anti-CD3-stimulated naive T cells (data not shown). These results indicate Mst1 is required for efficient Treg development in the thymus, but is not essential for peripheral Treg generation. T cell-dependent autoimmunity in Mst1-deficient mice Mst1-deficient mice spontaneously developed inflammatory infiltrates in multiple organs that increased with age and were accompanied by autoantibodies. One-year-old Mst1 −/− (CAG-Cre;Mst1 f/f ) mice exhibited leukocyte infiltration in the liver, lung, stomach ( Fig. 7a ), pancreas and kidney ( Supplementary Fig. S6a ). Tissue infiltrates were composed of CD3 + T cells, B220 + B cells, including plasmacytes, and CD11b + myeloid cells ( Supplementary Fig. S6b ). Autoantibodies to the tissues and double-strand DNA were also detected ( Fig. 7b,c ). T cell-specific Mst1-deficient mice ( lck-Cre;Mst1 f/f ) exhibited even more severe leukocyte infiltration and autoantibody production ( Fig. 7 ; Supplementary Fig. S6c ). In contrast, B cell-specific Mst1-deficient mice ( mb1-Cre; Mst1 f/f mice) did not develop apparent abnormalities for up to 18–20 months ( Fig. 7 ). 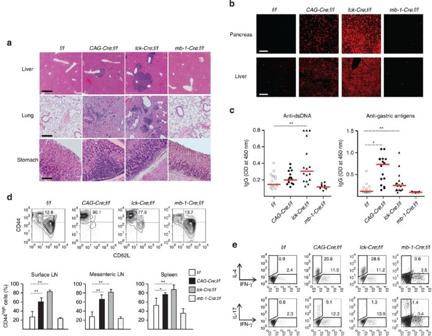Figure 7: Mst1-deficient mice develop autoimmune-like phenotypes. (a) Haematoxylin and eosin staining of paraffin sections of organs from 1-year-oldMst1f/f, CAG-Cre;Mst1f/f, lck-Cre;Mst1f/f, or mb1-Cre;Mst1f/fmice. Note that inflammatory infiltrates in the liver, lung and stomach inMst1f/f, CAG-Cre;Mst1f/f, lck-Cre;Mst1f/fmice. Scale bars represent 400 μm for liver, lung and 200 μm for stomach (b) Autoantibodies to tissues were detected in the sera of 1-year-oldMst1f/f, CAG-Cre;Mst1f/f, lck-Cre;Mst1f/f, or mb1-Cre;Mst1f/fmice by immunostaining with an anti-Igκ antibody (scale bar, 100 μm). (c) Titres of antibodies to double-stranded DNA (dsDNA) and stomach glandular epithelial cells in the serum ofMst1f/f,CAG-Cre;Mst1f/f,lck-Cre;Mst1f/for mb1-Cre;Mst1f/fmice. The bar in the graphs indicates the median.Pvalues were calculated by Mann–WhitneyU-test (d–f) *0.01<P<0.05; **P<0.01 (d) Expansion of effector–memory T cells inMst1−/−mice. The flow cytometric profiles of CD44 and CD62L among CD4+cells in the mesenteric lymph nodes of 1-year-oldMst1f/f, CAG-Cre;Mst1f/f, lck-Cre;Mst1f/for mb-1-Cre;Mst1f/fmice (upper panel). The bar graphs show the average percentages (±s.d.) of CD44hicells among CD4+T cells from various lymphoid tissues in 1-year-oldMst1f/f, CAG-Cre;Mst1f/f, lck-Cre;Mst1f/for mb-1-Cre;Mst1f/fmice (lower panel). (e) The increased production of effector cytokines in Mst1-deficient mice. Cytokine production by CD4+T cells from the mesenteric lymph node of 1-year-oldMst1f/f,CAG-Cre;Mst1f/f,lck-Cre;Mst1f/formb-1-Cre;Mst1f/fmice was measured by staining for intracellular IFN-γ, IL-4 and IL-17. Similar results were also obtained in peripheral lymphoid tissues. Figure 7: Mst1-deficient mice develop autoimmune-like phenotypes. ( a ) Haematoxylin and eosin staining of paraffin sections of organs from 1-year-old Mst1 f/f , CAG-Cre;Mst1 f/f , lck-Cre;Mst1 f/f , or mb1-Cre;Mst1 f/ f mice. Note that inflammatory infiltrates in the liver, lung and stomach in Mst1 f/f , CAG-Cre;Mst1 f/f , lck-Cre;Mst1 f/f mice. Scale bars represent 400 μm for liver, lung and 200 μm for stomach ( b ) Autoantibodies to tissues were detected in the sera of 1-year-old Mst1 f/f , CAG-Cre;Mst1 f/f , lck-Cre;Mst1 f/f , or mb1-Cre;Mst1 f/f mice by immunostaining with an anti-Igκ antibody (scale bar, 100 μm). ( c ) Titres of antibodies to double-stranded DNA (dsDNA) and stomach glandular epithelial cells in the serum of Mst1 f/f , CAG-Cre;Mst1 f/f , lck-Cre;Mst1 f/f or mb1-Cre;Mst1 f/f mice. The bar in the graphs indicates the median. P values were calculated by Mann–Whitney U -test ( d – f ) *0.01< P <0.05; ** P <0.01 ( d ) Expansion of effector–memory T cells in Mst1 −/− mice. The flow cytometric profiles of CD44 and CD62L among CD4 + cells in the mesenteric lymph nodes of 1-year-old Mst1 f/f , CAG-Cre;Mst1 f/f , lck-Cre;Mst1 f/f or mb-1-Cre;Mst1 f/f mice (upper panel). The bar graphs show the average percentages (±s.d.) of CD44 hi cells among CD4 + T cells from various lymphoid tissues in 1-year-old Mst1 f/f , CAG-Cre;Mst1 f/f , lck-Cre;Mst1 f/f or mb-1-Cre;Mst1 f/f mice (lower panel). ( e ) The increased production of effector cytokines in Mst1-deficient mice. Cytokine production by CD4 + T cells from the mesenteric lymph node of 1-year-old Mst1 f/f , CAG-Cre;Mst1 f/f , lck-Cre;Mst1 f/f or mb-1-Cre;Mst1 f/f mice was measured by staining for intracellular IFN-γ, IL-4 and IL-17. Similar results were also obtained in peripheral lymphoid tissues. Full size image Before the onset of apparent leukocyte infiltrates in multiple organs (2–3 months), increased activated effector–memory lymphocytes were detected in CAG-Cre;Mst1 f/f and lck-Cre;Mst1 f/f mice, and predominantly expanded in the peripheral lymphoid tissues by 1 year ( Fig. 7d ) with substantial increases of interferon (IFN)-γ-, interleukin (IL)-4- or IL-17-expressing CD4T cells in peripheral lymphoid tissues ( Fig. 7e ). To investigate whether the autoimmune phenotype that developed in Mst1 −/− mice could be due to impaired thymocyte selection, we adoptively transferred wild-type and Mst1 −/− thymocytes into T cell-deficient CD3ɛ −/− mice. After 10 weeks, the recipient mice invariably exhibited inflammatory infiltrates in multiple organs, including the liver, lung and stomach, whereas none of the control mice that received wild-type thymocytes developed this phenotype ( Fig. 8 ). To examine the role of LFA-1 and ICAM-1 in the selection process in vivo , we adoptively transferred thymocytes from ICAM-1-deficient mice into ICAM-1-sufficient CD3ɛ −/− mice. We used thymocytes from ICAM-1-deficient mice as LFA-1 is required for peripheral T-cell trafficking and effector functions. Thymocytes from ICAM-1 −/− mice, but not wild-type mice, caused inflammatory infiltrates in the liver, lung and stomach at 10 weeks after adoptive transfer ( Fig. 8 ). 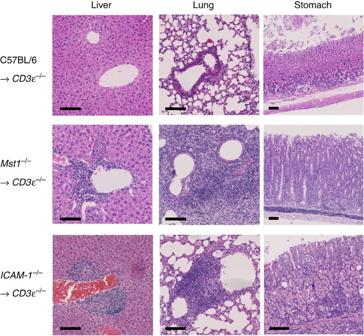Figure 8: Adoptive transfer ofMst1−/−andICAM-1−/−thymocytes induces inflammation. Haematoxylin and eosin staining of tissue sections from the lung, stomach and liver ofCD3ɛ−/−mice 10 weeks after adoptively transferring 3−5×107thymocytes from C57BL/6,Mst1−/−orICAM-1−/−mice (C57BL/6,n=6;Mst1−/−,n=4;ICAM-1−/−,n=4). Inflammatory infiltrates in the liver, lung and stomach in mice transferred withMst1−/−orICAM1−/−thymocytes are present in all cases, but none with wild-type thymocytes. Representative images are shown. Scale bar, 100 μm. Figure 8: Adoptive transfer of Mst1 −/− and ICAM-1 −/− thymocytes induces inflammation. Haematoxylin and eosin staining of tissue sections from the lung, stomach and liver of CD3ɛ −/− mice 10 weeks after adoptively transferring 3−5×10 7 thymocytes from C57BL/6, Mst1 −/− or ICAM-1 −/− mice (C57BL/6, n =6; Mst1 −/− , n =4; ICAM-1 −/− , n =4). Inflammatory infiltrates in the liver, lung and stomach in mice transferred with Mst1 −/− or ICAM1 −/− thymocytes are present in all cases, but none with wild-type thymocytes. Representative images are shown. Scale bar, 100 μm. Full size image Collectively, these data suggest that Mst1 regulation of thymocyte adhesion and migration through LFA-1 and ICAM-1 has crucial roles in the thymocyte selection process. Using the thymic slice method, we demonstrated that an Mst1 deficiency or blocking LFA and ICAM-1 impaired T cell intrinsic processes in medullary migration and recognition of self-antigen on Aire + mTECs. Mst1-deficient mice developed T cell-dependent autoimmune phenotypes with age. These results suggest that Mst1 is required for efficient negative selection in the medullary region by controlling thymocyte trafficking through LFA-1. The Mst1-dependent high motility of mature SP cells is likely required for efficient scanning of very small numbers of Aire + ICAM-1 + mTECs expressing TRA during their limited resident time (4−5 days) in the medulla [35] . This study identified a previously unrecognized role for LFA-1 and ICAM-1 in these processes and suggests that Mst1 has an important role in integrin regulation to establish self-tolerance in the thymus. Previous studies demonstrated that SP cells migrate faster than DP cells [10] , [11] . This study demonstrated that thymic environment abundantly expresses ICAM-1, especially in the medulla and support the high-velocity migration of SP cells via LFA-1. SP cells, unlike DP cells, migrate rapidly on ICAM-1 with chemokine signalling. Interestingly, it was shown previously that Rap1 was activated in positively selected thymocytes [36] . This suggests that Rap1 signalling to Mst1 is acquired after positive selection and enables selected thymocytes to migrate to the medulla [8] through integrin activation. Mst1 deficiency affected the number of CD69 + SP cells. The trafficking patterns of DP and the number of immature positively selected CD69 + DP in Mst1 −/− mice were comparable to those of wild type, suggesting that antigen scanning of DP in the cortex is intact. The decrease in mature CD69 + SP cells in Mst1 −/− mice might be due to impaired trafficking of positively selected SP thymocytes to the medulla. OT-II SP exhibited arrest rather than transient contact with Aire + mTECs, leading to cluster formations in several hours, suggesting that the high expression of ICAM-1 by Aire + mTEC is likely instrumental in efficient recognition of self-antigen presented by mTEC. The clusters were dissociated with increased velocities by 24 h. These dynamic behaviours of SP cells were reminiscent of those of peripheral naive T cells interacting with antigen-presenting DC [37] , [38] . The previous study with the OT-I/RIP-mOVA system showed that negatively selected thymocytes moved relatively slowly and made frequent, brief contacts with surrounding DC [10] . Because this study used the partial BM chimera, generation of mature thymocytes is not synchronized. As mTEC was not visualized in this study, it would be difficult to detect the point at which mature thymocytes are arrested when they encountered negatively selecting ligands presented on mTEC. A brief contact of SP cells with CD11c + DC may represent distinct steps of negative selection. Autoreactive OVA-specific thymocytes are negatively selected in RIP-mOVA mice, which require Aire expression [6] . We demonstrated that Aire + mTEC could provide SP cells with negatively selecting ligands to trigger calcium influx and strong adhesive interactions with SP cells via LFA-1 and ICAM-1. Based on the tight association of OT-II SP cells with Aire + mTEC, it is interesting to speculate that Aire + mTEC could be the site of negative selection. This notion is consistent with the finding that mTEC can mediate tolerance by direct presentation of Aire-regulated antigens to both CD4 and CD8 T cells [30] . Treg development in the thymus requires strong peptide–MHC interaction [39] and CD18 (ref. 40 ), and may share the same mTEC with CD4SP cells [41] . Mst1 −/− CD4SP cells exhibited decreased contact frequency and stable association with cognate Aire + ICAM-1 + mTEC. These results suggest the importance of LFA-1/ICAM-1-dependent interactions regulated by Mst1 for negative selection and Treg generation. The frequency of antigen recognition by SP cells is influenced by migration velocities, adhesion strength to APC and resident time in the medulla. These factors of trafficking are critical for efficient removal of autoreactive SP cells, especially when the probability of SP cells to encounter cognate antigen is extremely limited; one TRA is only expressed by 0.5–2% of mTECs [3] and the frequency of SP cells specific for the TRA is also very low in normal polyclonal repertoire. Despite inefficient antigen recognition by Mst1 −/− SP cells, the impairment of negative selection process of Mst1 −/− mice were relatively mild in transgenic models, perhaps due to abundant self-antigen and fixed TCR. We showed that impaired self-tolerance was induced by Mst1 −/− or ICAM-1 −/− thymocyte transfer, indicating that defective migration of SP cells by Mst1 or ICAM-1 deficiency actually affect elimination of autoreactive thymocytes in non-transgenic conditions. Regarding the cause–effect relationship of thymocyte egress and selection, it is unlikely that the defective thymocyte egress directly impair selection processes, as in S1P1-deficient mice immature DP and CD62L lo SP cells were not changed [42] , and there are no definitive reports on impaired thymocyte selection in S1P1 −/− mice, or in mice administered with S1P inhibitors. Mst1 −/− SP cells exhibited intact or mild affected chemotactic response to S1P, whereas CCL21/CCL19-dependent chemotaxis or migration on ICAM-1 was more severely affected [21] , [23] (this study). We speculate that defective migration of mature Mst1 −/− thymocytes triggered with chemokines and integrin ligands also affect egress processes. The roles of LFA-1 and ICAM-1 in thymocyte selection process have not been previously recognized. A complete loss of LFA-1 leads to immunodeficiency and inhibits the development of autoimmunity. Adoptive transfer of ICAM-1-deficient thymocytes into ICAM-1-sufficient hosts resulted in impaired central tolerance, suggesting a requirement of functional LFA-1 in periphery to develop the autoimmunity. Inside-out signalling that regulates integrins is mediated by multiple pathways [43] . The impaired integrin regulatory pathway by Mst1 deficiency could perturb self-tolerance, but not development of the autoimmunity, suggesting that Mst1 is more critical as an inside-out signal in thymocytes and naive lymphocytes rather than activated effector cells. Thus, this study provides an insight into the roles of LFA-1 in thymic selection and autoimmune disorders. Mice Mst1 flox/flox mice on a C57BL/6 background were previously described [20] . C57BL/6 mice were purchased from Clea, Japan. OT-II, RIP-mOVA, CD11c-EYFP, and ECFP transgenic mice and ICAM -1 −/− mice on a C57BL/6 background were obtained from Jackson Laboratories. CAG-Cre transgenic mice and H-Y TCR transgenic mice were kindly provided by Dr S. Yamada (Akita University, Akita, Japan) and Dr S. Sakaguchi (Osaka University, Osaka, Japan). Lck-Cre and mb1-Cre transgenic mice were obtained from Animal Resources and Development at Kumamoto University (Kumamoto, Japan). CD3ɛ −/− , Ly5.1 mice were kindly provided by Dr M. Hori (RIKEN, Yokohama, Japan). Aire-GFP knock-in mice were previously described [44] . All mice were maintained under specific pathogen-free conditions in the animal facility at Kansai Medical University. All animal experiments were in accordance with protocols approved by the Animal Care and Use Committee of Kansai Medical University (Osaka, Japan). Antibodies and reagents FITC-, PE-, PE-Cy7-, PerCP-Cy5.5-, Alexa Fluor 647-, APC-, APC-eFluor-780- or eFluor 450-labelled antibodies specific to Aire, B220, CD3, CD4, CD8, CD11a, CD11b, CD11c, CD24, CD31, CD44, CD45.1, CD45.2, CD54, CD62L, CD138, FoxP3, Gr-1, Igκ, IFN-γ, IL-4, IL-7, T3.70, TCR-β, Vα2 and Vβ5 were from BD Biosciences or eBioscience. Anti-Foxo1 and Foxo3 were from Cell Signaling Technologies. Rabbit keratin 5 antibodies were from Covance. Antibody concentrations for immunohistchemistry and flow cytometry were at 0.1–5 μg ml −1 . Staining of CCR7 was described [45] . FITC-labelled PNA and UEA-1 were obtained from Vector Laboratories (Burlingame, CA). Cy5-labelled AnnexinV (1:100 dilution) was purchased from Biovision (Milpitas, CA). Alexa Fluor 488-, 546-, 633- or FITC-conjugated goat anti-mouse, anti-rat, anti-rabbit or anti-human IgG (1–2 μg ml −1 ) from Jackson ImmunoResearch Laboratories, Invitrogen or ICN Biomedicals were used. CFSE (5- or 6-( N -succinimidyloxycarbonyl)-fluorescein 3′,6′-diacetate), CMTMR ((5-(and 6)-(((4-chloromethyl)benzoyl)amino) tetramethylrhodamine) dye and Indo-PE3-AM (2 μg ml −1 ) for cell labelling were obtained from Invitrogen or TEFLabs. Thymic slice preparation and imaging by two-photon microcopy Preparation of thymic slices and imaging using a two-photon laser microscope were performed as described [9] with some modifications. A thymic lobe was embedded on a handmade plastic pedestal with low-melting agarose (Sigma-Aldrich). The thymic slice was cut every 400 μm using a vibratome (DSK, Kyoto, Japan), and incubated with complete medium (RPMI-1640 containing 8% FCS, 50 μM 2-mercaptoethanol, 10 mM HEPES and antibiotics) for a few minutes at room temperature. The slices were placed onto a Millicell insert (30-mm organotypic PTFE; Millipore) in a 3.5-mm plastic Petri dish filled with 1 ml complete medium and then enclosed using silicone grease. The thymocytes were labelled with either 1 μM CFSE or 1 μM CMTMR (Invitrogen) in 1 ml per 1×10 7 of RPMI-1640 containing 1% FCS for 25 min at 37 °C. The labelled thymocytes (DP: 0.5−1×0 6 , SP: 1×10 5 ) were suspended in complete medium and loaded onto slices, and the cells on the slice were incubated for 3−24 h at 37 °C/5% CO 2 to allow cells to enter the tissue. For calcium imaging, thymocytes were labelled with 2 μM of Indo-PE3 (TEFLabs) for 30 min and layered onto thymic slices. The incubated thymic slice was placed on handmade plastic pedestal using a tissue adhesive (Vetbond; 3 M). Then, the slices were mounted on the bottom of a RC-26 flow chamber (Warner Instruments) using silicone grease. Pre-warmed RPMI-1640 medium bubbled with 95% O 2 and 5% CO 2 continuously flowed over the slice at a rate of 1–2 ml min −1 . The temperature was maintained at 36−37 °C using both the chamber and an in-line heater. Two-photon imaging was performed using a FV1000 upright microscope (Olympus), with a Ti:sapphire laser (MaiTai HP DeepSee-OL, Spectra-Physics) tuned to 850 nm (or 900 nm for EGFP) and a X25/1.05 NA objective (XLPLN25XWMP, Olympus). Emitted light was passed through 495−540 nm and 575−630 bandpass filters to photomultiplier (PMT) for detection of CFSE (EGFP) and CMTMR fluorescence. In some cases, excitation at 820 nm with bandpass filters 460−500 nm, 520−560 nm and 575−630 nm was used for detection of enhanced cyan fluorescent protein (ECFP), CFSE and CMTMR, respectively. Acquisition was controlled with FV10-ASW software (Olympus), and Z stacks were typically acquired every 15−20 s, with Z steps spaced 2−2.5 μm apart. Imaging was performed 10−200 μm beneath the cut surface of the slice. Volocity (Improvison) was used for tracking cell positions over time in three dimensions. Image stack sequences were transformed into volume-rendered four-dimensional movies. From the x , y , z coordinates of cell centroids, cellular motility parameters were calculated as described [37] . To detect Indo-PE3-labelled thymocytes, samples were excited with 710 nm and the emitted fluorescence was split with a 440-nm dichroic filter and passed through 390/70 (Ca 2+ bound) and 465−565 bandpass filters (Ca 2+ unbound). The ratio of Ca 2+ bound/Ca 2+ unbound was calculated and analysed using Volocity software (Perkin-Elmer, Waltham, MA). Two-dimensional migration assay Recombinant mouse ICAM-1-Fc was used to coat pre-washed glass-bottom dishes, as described [46] with or without 100 nM CCL21 (R&D systems). Thymocytes were stained with anti-CD8-PE, and CD4 + SP thymocytes were negatively enriched using magnetic cell sorting with anti-PE-beads (Miltenyi Biotec). The enriched thymocytes were labelled with CFSE and CMTMR, suspended in L-15 medium (Sigma-Aldrich) containing 5% FCS and loaded onto pre-warmed ICAM-coated dishes on a temperature-controlled stage. Time-lapse imaging was acquired every 10 s using a confocal microscope with 488- and 543-nm lasers with Metamorph software (Molecular Devices). Adhesion assays Adhesion assays using recombinant mouse ICAM-1Fc proteins were performed as described [20] . After blocking with 1% BSA, CD4SP cells isolated by magnetic-activated cell sorting (MACS) were labelled with 2′,7′-bis-(2-carboxyethyl)-5-(and-6)-carboxyfluorescein, acetoxymethyl ester (Molecular Probes), and incubated on an ICAM-1-coated 96-well plate (1×10 5 cells per well) with or without anti-CD3 (145-2C11, 10 μg ml −1 ) at 37 °C for 30 min. Non-adherent cells were removed by four consecutive washes. Fluorescence of input and bound cells in triplicates were measured with a fluorescence plate reader (Cyotofluor4000, Applied Biosystems) and calculated percentages of bound cells. Cell sorting Isolated thymocytes were stained with antibodies to mouse CD4 (0.003 μg ml −1 ), CD8 (0.01 μg ml −1 ) or CD69 (0.4 μg ml −1 ) and thymocyte subsets were sorted using a FACSAria I Cell Sorter. To avoid cell damage, the sorting conditions were optimized with a low pressure of 10 psi with 100-μm diameter nozzles. Wild-type and OT-II CD4 + thymocytes were stained with an anti-CD8-PE antibody (0.02 μg ml −1 ) and sorted by cell sorter. Alternatively, anti-CD8-PE (0.1 μg ml −1 )-stained thymocytes were then incubated with anti-PE magnetic beads (Miltenyi Biotec). Then, CD4 + SP thymocytes were negatively enriched (70−80%) using magnetic cell sorting (Miltenyi Biotec). Adoptive reconstitutions (C57BL/6×C57BL/6.CD45.1)F1 mice were lethally irradiated (950 rad) and reconstituted with equal numbers (5×10 6 ) of congenic C57BL/6.CD45.1 and Mst1 −/− BM cells to generate mixed chimeric mice. In some experiments, (RIP-mOVA×C57BL/6.CD45.1)F1 were reconstituted with a mixture of T cell-depleted BM cells from (C57BL/6×C57BL/6.CD45.1)F1 OT-II and Mst1 −/− OT-II BM cells. The donor and recipient cells in the chimeras were distinguished based on CD45.1 and CD45.2 expression. Chimerism in the BM and thymus was determined based on the CD45.1/CD45.2 ratio. The efficiency of reconstitution in Mst1 −/− thymocytes was only ∼ 10% of that in wild-type thymocytes. Therefore, to control for any effects of hematopoietic reconstitution, mixed chimeric mice with CD45.1 and wild-type BM cells (9:1) were also generated. Immunohistochemistry Cryostat sections of frozen tissues (10 μm) were fixed with acetone, air-dried and stained with the indicated antibodies. To detect tissue-binding autoantibodies, diluted (×100) serum samples were loaded onto tissue sections for 1 h, and then detected using a rat anti-mouse Igκ-PE antibody or anti-mouse IgG FITC F(ab) 2 fragments (3 μg ml −1 ). Images of stained sections were acquired using a confocal microscope (LSM510-META, Zeiss). Histology Organs from mice were collected and fixed overnight in 10% formalin, embedded in paraffin, sectioned and stained with haematoxylin and eosin (H&E). Digital images of organs were acquired by Nanozoomer (Hamamatsu Photonics). Flow cytometry Cells (0.5–2.×10 6 ) were stained with antibody cocktails that visualize T cell, B cell, myeloid cells, plasmacytes or thymocyte subsets, respectively. Stained cells are analysed by either FACS calibre or FACS Canto II flow cytometer (BD Bioscience). Dead cells were excluded by gating live cell size and/or gating out of propidium iodide (Sigma-Aldrich) stained cells. Intracellular cytokine staining A range of 0.5−2.×10 6 cells were stimulated with phorbol myristate acetate (50 ng ml −1 )+ionomycin (1 μg ml −1 ) for 4 h. Then, the cells were collected, fixed and permeabilized with BD Cytofix/Cytoperm Fixation/Permeabilization Solution Kit (BD Biosciences), followed by staining with antibodies to IFN-γ, IL-4 and/or IL-17 (1 μg ml −1 ; eBioscience) at room temperature for 20 min. ELISA ELISA assays for anti-stomach antibodies present in the serum (diluted 40-fold) were performed using total microsomal fractions extracted from the glandular stomachs [47] as antigen. Similarly, anti-double-stranded DNA antibodies were measured using calf thymus DNA (Sigma-Aldrich) treated with S1-nuclease (Invitrogen). Antibody binding was detected using HRP-conjugated anti-mouse IgG (1:8,000; Southern Biotech) with TMB substrate (eBioscience). Serum from 6-month-old MRL.lpr/lpr mice was used as a positive control. Western blotting CD4SP from thymocytes were isolated by cell sorting, and lysed with lysis buffer (1% TritonX-100, 50 mM Tris–HCl pH 8.0, 150 mM NaCl, 1 μg ml −1 aprotinin, 1 mM phenylmethylsulphonyl fluoride). Cell lysates were subjected to immunoblotting [20] . Statistical analysis Student's t -test was performed if the data were normally distributed. Otherwise, Mann−Whitney U -test was performed. To analyse the chimeric mice, paired Student's t -test was used. How to cite this article: Ueda, Y. et al . Mst1 regulates integrin-dependent thymocyte trafficking and antigen recognition in the thymus. Nat. Commun. 3:1098 doi: 10.1038/ncomms2105 (2012).